IRF8 suppresses pathological cardiac remodelling by inhibiting calcineurin signalling Interferon regulatory factor 8 (IRF8) is known to affect the innate immune response, for example, by regulating the differentiation and function of immune cells. However, whether IRF8 can influence cardiac hypertrophy is unknown. Here we show that IRF8 levels are decreased in human dilated/hypertrophic cardiomyopathic hearts and in murine hypertrophic hearts. Mice overexpressing Irf8 specifically in the heart are resistant to aortic banding (AB)-induced cardiac hypertrophy, whereas mice lacking IRF8 either globally or specifically in cardiomyocytes develop an aggravated phenotype induced by pressure overload. Mechanistically, we show that IRF8 directly interacts with NFATc1 to prevent NFATc1 translocation and thus inhibits the hypertrophic response. Inhibition of NFATc1 ameliorates the cardiac abnormalities in IRF8 −/− mice after AB. In contrast, constitutive activation of NFATc1 nullifies the protective effects of IRF8 on cardiac hypertrophy in IRF8-overexpressing mice. Our results indicate that IRF8 is a potential therapeutic target in pathological cardiac hypertrophy. Heart failure is among the most prevalent causes of mortality globally. A major risk factor for heart failure development is cardiac hypertrophy, which has various causes, including hypertension, myocardial infarction, valvular heart disease and endocrine disorders [1] , [2] . Despite extensive studies, the mechanisms controlling the progression from adaptive hypertrophy to heart failure remain poorly understood. Cardiac hypertrophy results from a complex signalling cascade involving the MAPK, PI3K/Akt, PKC, NFκB, cAMP-response element binding protein (CREB) and calcineurin/nuclear factor of activated T cells (NFAT) pathways [3] , [4] , [5] , [6] . Multiple signalling cascades converge upon certain transcription factors, activating nuclear cardiac fetal gene programs and ultimately leading to pathological cardiac hypertrophy [4] , [7] . Therefore, molecules that selectively affect the activity of specific transcription factors could be of great therapeutic interest for treating cardiac hypertrophy. Interferon regulatory factor 8 (IRF8), also known as interferon consensus sequence-binding protein, is a member of the IRF family of transcription factors that are induced by interferon in a variety of cell types [8] . IRF8 itself is induced by interferon in macrophages and T cells, with its induction mediated by a gamma activation sequence element in the IRF8 promoter [9] , [10] , [11] . IRF8 exerts its activity through the formation of different DNA-binding heterocomplexes with multiple partners, including members of the IRF family (IRF1, IRF2 and IRF4) and non-IRF transcription factors (PU.1, TEL, E47 and MIZ1) [12] , [13] . Once expressed, IRF8 either activates or represses the transcription of downstream target genes, which are dependent upon their interacting partners [14] , [15] . A large number of studies have demonstrated that IRF8 functions as a transcription factor in the regulation of the innate immune response and plays critical roles in the differentiation of myeloid cells [15] , [16] , while IRF8 also could function as a regulator factor to regulate innate and adaptive immune responses and other biological processes [17] , [18] , [19] . In addition, IRF8 has been implicated as a tumour suppressor gene in certain hematopoietic cancers and solid tumour [20] , [21] . Interestingly, an increasing number of studies have supported the involvement of tumour suppressors in negatively modulating cardiac hypertrophy [22] , [23] , raising the possibility that IRF8 might regulate cardiac hypertrophy. However, the role of IRF8 in cardiac hypertrophy has not yet been studied and remains uncharacterized. Therefore, the aims of the current study were as follows: first, to determine whether IRF8 is altered in human dilated cardiomyopathy (DCM) hearts, in human hypertrophic cardiomyopathy (HCM) hearts and in an animal model of cardiac hypertrophy induced by pressure overload; second, to determine whether IRF8 might affect cardiac hypertrophy; finally, if so, to determine the responsible mechanisms involved. Here we show that IRF8 is downregulated in both mouse hearts and cardiomyocytes after hypertrophic stress treatment. Moreover, IRF8-deficient mice reveal an aggravated pressure overload-induced hypertrophic response, whereas the opposite effects occur in IRF8-overexpressing mice. We also report that the IAD1 domain of IRF8 (N/200–377aa) could interact with the TAD-A domain (N/1-205aa) of NFATc1 to inhibit the nuclear translocation of NFATc1. Furthermore, inhibition of NFATc1 with a cell-permeable NFAT inhibitory peptide (VIVIT) counter acts the effects of IRF8 deficiency, whereas constitutively active NFATc1 (CaNFATc1) negates the anti-hypertrophic effects of IRF8. Taken together, our results indicate that IRF8 is a novel negative regulator of pathological cardiac hypertrophy, largely via its interaction with NFATc1. IRF8 expression is decreased in hypertrophic hearts To explore the potential role of IRF8 in the development of cardiac hypertrophy and heart failure, we first examined whether the IRF8 expression levels were altered in pathological hearts. Western blotting and real-time polymerase chain reaction (PCR) revealed that the IRF8 messenger RNA (mRNA) and protein expression levels were significantly decreased in DCM human hearts, compared with donor hearts ( Fig. 1a,b and Supplementary Fig. 1a ). IRF8 reduction was accompanied by an upregulation in the expression of cardiac hypertrophic markers, that is, atrial natriuretic peptide (ANP), β-myosin heavy chain (β-MHC) ( Fig. 1a,b and Supplementary Fig. 1b ), which was consistent with the results of HCM hearts ( Fig. 1c,d ). In an experimental mouse model of aortic banding (AB)-induced cardiac hypertrophy (as evidenced by elevated levels of β-MHC and ANP, Fig. 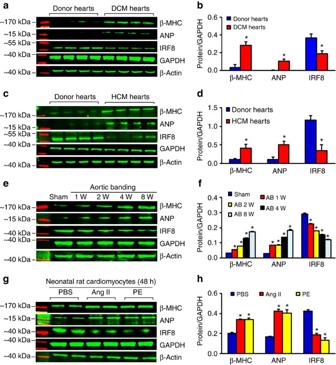Figure 1: IRF8 Expression is decreased in DCM/HCM human hearts and in hypertrophic murine hearts. (a,b) a, Representative western blots; b, quantitative results of β-MHC, ANP and IRF8 protein expression in donor hearts and in DCM hearts (n=6 samples per experimental group, *P<0.05 versus donor). (c,d) c, Western blot analysis; d, quantitative results of β-MHC, ANP and IRF8 protein expression in HCM hearts and in donor hearts (n=4 samples per experimental group, *P<0.05 versus donor). (e,f) e, Western blot analysis; f, quantitative results of β-MHC, ANP and IRF8 protein expression in a mouse model of cardiac hypertrophy induced by AB for the indicated time (n=4 mice per experimental group, *P<0.05 versus sham). (g,h) g, Representative western blots; h, quantitative results of β-MHC, ANP and IRF8 protein expression in NRCMs treated with Ang II (1 μM) or PE (100 μM) for 48 h (n=4 samples per experimental group, *P<0.01 versus PBS). The data represent as the mean±s.d. Statistical analysis was carried out by Student’s two-tailedt-test. 1e,f ), IRF8 levels were progressively downregulated by ~38% in mouse hearts at week 2 after AB, by ~46% at week 4 after AB and by ~57% at week 8 after AB, compared with sham-operated hearts ( Fig 1e,f , n =3 independent experiments, P< 0.05 versus Sham; statistical analysis by Student’s two-tailed t- test). The immunofluorescence results showed that IRF8 was expressed in both the cytoplasm and nucleus of cardiomyocytes and that its expression was downregulated in hypertrophic hearts ( Supplementary Fig. 1c ). Furthermore, using in vitro cultured neonatal rat cardiomyocytes (NRCMs) treated with either angiotensin II (Ang II, 1 μM) or phenylephrine (PE, 100 μM) for 48 h to induce hypertrophy, we found that IRF8 expression was also reduced by ~55% (Ang II) and ~68% (PE) in these hypertrophic cardiomyocytes ( Fig. 1g,h , n =3 independent experiments, P< 0.01 versus phosphate-buffered saline (PBS); statistical analysis by Student’s two-tailed t- test).Thus, IRF8 is significantly decreased in DCM/HCM human hearts and in pressure overload-induced hypertrophic murine hearts as well as in in vitro Ang II/PE-treated cardiomyocytes. Figure 1: IRF8 Expression is decreased in DCM/HCM human hearts and in hypertrophic murine hearts. ( a , b ) a, Representative western blots; b, quantitative results of β-MHC, ANP and IRF8 protein expression in donor hearts and in DCM hearts ( n =6 samples per experimental group, * P< 0.05 versus donor). ( c , d ) c, Western blot analysis; d, quantitative results of β-MHC, ANP and IRF8 protein expression in HCM hearts and in donor hearts ( n =4 samples per experimental group, * P< 0.05 versus donor). ( e , f ) e, Western blot analysis; f, quantitative results of β-MHC, ANP and IRF8 protein expression in a mouse model of cardiac hypertrophy induced by AB for the indicated time ( n =4 mice per experimental group, * P< 0.05 versus sham). ( g , h ) g, Representative western blots; h, quantitative results of β-MHC, ANP and IRF8 protein expression in NRCMs treated with Ang II (1 μM) or PE (100 μM) for 48 h ( n =4 samples per experimental group, * P< 0.01 versus PBS). The data represent as the mean±s.d. Statistical analysis was carried out by Student’s two-tailed t- test. Full size image IRF8 suppresses Ang II-induced cardiomyocyte hypertrophy Decreased IRF8 expression in response to hypertrophic stimuli implies a potential role for IRF8 in the regulation of pathological cardiac hypertrophy. To test this hypothesis, we performed gain- and loss-of-function studies in NRCMs. NRCMs were infected with either AdshIRF8 to knockdown IRF8 or AdIRF8 to overexpress IRF8 ( Supplementary Fig. 2 ). The cells were then stimulated with Ang II (1 μM) or PBS control for 48 h and were immunostained with α-actinin for cellular size measurement. The IRF8 deficiency mediated by AdshIRF8 infection remarkably increased Ang II-induced cardiomyocyte hypertrophy, whereas IRF8 overexpression by AdIRF8 significantly inhibited cell hypertrophy (as evidenced by cardiomyocyte cell surface area, Fig. 2a,b ). The levels of hypertrophic markers (ANP and β-MHC) were increased during IRF8 knockdown, and decreased during IRF8 overexpression ( Fig. 2c ). These data implicate IRF8 as a negative regulator of cardiac hypertrophy. 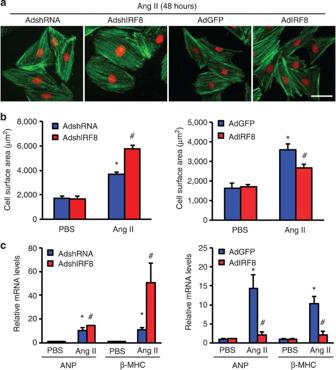Figure 2: IRF8 protects against Ang II-induced cardiomyocyte hypertrophyin vitro. (a) Representative images of cardiomyocytes infected with AdshIRF8 or AdIRF8 and treated with Ang II (1 μM) for 48 h (red: nuclear; green: α-actinin; scale bar, 50 μm). (b) Quantitative results of the cell surface area of cardiomyocytes infected with AdshIRF8 or AdIRF8 in response to Ang II (1 μM) for 48 h (n≥50 cells per experimental group). (c) Real-time PCR assays were performed to determine the mRNA levels of ANP and β-MHC in IRF8 knockdown and overexpressed cells after treatment with PBS and Ang II for 48 h. (n=4 samples per experimental group, *P<0.05 versus AdshRNA or AdGFP /PBS, #P<0.05 versus AdshRNA or AdGFP /Ang II). The data represent as the mean±s.d. Statistical analysis was carried out by two-way analysis of variance with general linear model procedures using a univariate approach. Figure 2: IRF8 protects against Ang II-induced cardiomyocyte hypertrophy in vitro. ( a ) Representative images of cardiomyocytes infected with AdshIRF8 or AdIRF8 and treated with Ang II (1 μM) for 48 h (red: nuclear; green: α-actinin; scale bar, 50 μm). ( b ) Quantitative results of the cell surface area of cardiomyocytes infected with AdshIRF8 or AdIRF8 in response to Ang II (1 μM) for 48 h ( n ≥50 cells per experimental group). ( c ) Real-time PCR assays were performed to determine the mRNA levels of ANP and β-MHC in IRF8 knockdown and overexpressed cells after treatment with PBS and Ang II for 48 h. ( n =4 samples per experimental group, * P< 0.05 versus AdshRNA or AdGFP /PBS, # P< 0.05 versus AdshRNA or AdGFP /Ang II). The data represent as the mean±s.d. Statistical analysis was carried out by two-way analysis of variance with general linear model procedures using a univariate approach. Full size image IRF8 deletion aggravates AB-induced hypertrophy To evaluate the anti-hypertrophic effects of IRF8 in vivo , we first utilized a mouse model with a global knockout of IRF8 (IRF8 −/− ), in which IRF8 cardiac expression was absent ( Supplementary Fig. 3a ). Notably, at baseline, IRF8 −/− mice manifested no pathological alterations in cardiac structure or function ( Supplementary Table 1 ). Furthermore, to clarify the effects of aging on the cardiac function of IRF8 −/− mice, we also assessed the phenotypes of cardiac function and structure in 47-week-old IRF8 −/− and wild-type (IRF8 +/+ ) mice. The results showed no significant differences in heart weight (HW)/body weight (BW), HW/tibia length (TL) and lung weight (LW)/BW, cross sectional area, collagen volume or echocardiography (LV end-diastolic dimension (LVEDD), LV end-systolic dimension (LVESD), fraction shortening (FS%)) between IRF8 −/− and IRF8 +/+ mice ( Supplementary Fig. 3b–f ). However, 2 weeks after AB, IRF8 −/− mice exhibited a remarkable deterioration in cardiac hypertrophy compared with IRF8 +/+ mice, as indicated by increased ratios of HW/BW, LW/BW and HW/TL ( Fig. 3a–c ). Histological examination revealed increased cross sectional area of cardiomyocytes in IRF8 −/− mice compared with IRF8 +/+ mice after a 2-week course of AB ( Fig. 3d,e ). Accordingly, the mRNA levels of several hypertrophic markers, including ANP, BNP and β-MHC, were much higher in IRF8 −/− mice than in IRF8 +/+ mice 2 weeks after AB ( Supplementary Fig. 3h ). Additionally, echocardiographic and hemodynamic measurements demonstrated that IRF8 deficiency significantly exacerbated AB-induced cardiac dilation and dysfunction compared with control IRF8 +/+ mice ( Fig. 3f and Supplementary Table 2 ). Accordingly, the cumulative survival rate was decreased in IRF8 knockout mice 2 weeks after AB surgery compared with controls ( Supplementary Fig. 3g ). 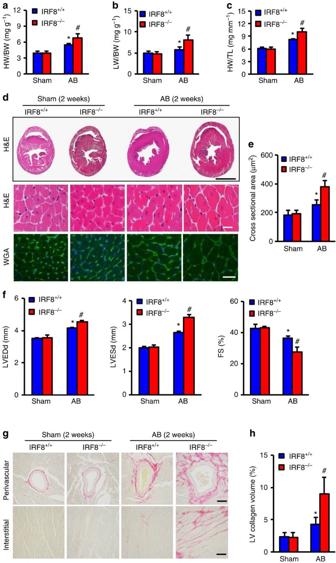Figure 3: IRF8 deficiency aggravates pressure overload-induced hypertrophy. (a–c) Statistical results for the ratios of (a) HW/BW, (b) LW/BW and (c) HW/TL in the indicated groups (n=11–13 mice per experimental group). (d) Histological analyses of the HE staining and WGA staining of IRF8+/+and IRF8−/−mice 2 weeks after AB surgery (n=6 mice per experimental group; scale bar, 100 μm for upper HE staining, scale bar, 20 μm for lower HE staining and WGA staining). (e) Statistical results for the cell sectional area (n≥100 cells per experimental group). (f) Parameters of the echocardiographic results for IRF8+/+and IRF8−/−mice (n=5–6 mice per experimental group). (g) PSR staining on histological sections of the heart in the indicated groups 2 weeks after AB (n=6 mice per experimental group; scale bar, 50 μm). (h) Statistical results for LV collagen volume (n≥40 fields per experimental group). *P<0.05 versus IRF8+/+/sham; #P<0.05 versus IRF8+/+/AB. The data represent as the mean±s.d. Statistical analysis was carried out by two-way analysis of variance with general linear model procedures using a univariate approach. Figure 3: IRF8 deficiency aggravates pressure overload-induced hypertrophy. ( a – c ) Statistical results for the ratios of ( a ) HW/BW, ( b ) LW/BW and ( c ) HW/TL in the indicated groups ( n =11–13 mice per experimental group). ( d ) Histological analyses of the HE staining and WGA staining of IRF8 +/+ and IRF8 −/− mice 2 weeks after AB surgery ( n =6 mice per experimental group; scale bar, 100 μm for upper HE staining, scale bar, 20 μm for lower HE staining and WGA staining). ( e ) Statistical results for the cell sectional area ( n ≥100 cells per experimental group). ( f ) Parameters of the echocardiographic results for IRF8 +/+ and IRF8 −/− mice ( n =5–6 mice per experimental group). ( g ) PSR staining on histological sections of the heart in the indicated groups 2 weeks after AB ( n =6 mice per experimental group; scale bar, 50 μm). ( h ) Statistical results for LV collagen volume ( n ≥40 fields per experimental group). * P< 0.05 versus IRF8 +/+ /sham; # P< 0.05 versus IRF8 +/+ /AB. The data represent as the mean±s.d. Statistical analysis was carried out by two-way analysis of variance with general linear model procedures using a univariate approach. Full size image We next assessed AB-induced cardiac fibrosis, a classical feature of the development of pathological cardiac hypertrophy. Paraffin-embedded slides were stained with picrosirius red (PSR) to determine the extent of fibrosis. Both interstitial and perivascular fibrosis were markedly increased in AB-treated IRF8 +/+ hearts but to a more prominent extent in IRF8 −/− hearts 2 weeks after AB ( Fig. 3g ). Cardiac fibrosis was further quantified by measuring the left ventricular (LV) collagen volume and the expression of the fibrotic markers Collagen I, Collagen III and connective tissue growth factor (CTGF) and revealed that the AB-induced fibrotic response was significantly activated in IRF8 −/− mice compared with IRF8 +/+ mice ( Fig. 3h and Supplementary Fig. 3i ). Collectively, these loss-of-function data indicate that IRF8 deficiency aggravates the pathological cardiac remodelling induced by chronic AB. To define specifically the effects of IRF8 on the heart, we generated a mouse model with a cardiac-specific deletion of IRF8 by crossing IRF8-Flox mice (B6(Cg)-Irf8 tm1.1Hm /J, Jackson Laboratory, 014175) with mice carrying the α-myosin heavy chain (α-MHC)–MerCreMer transgene (MEM-Cre-Tg (Myh6-cre/Esr1), Jackson Laboratory, 005650), as shown in Supplementary Fig. 4a–c . Cardiac-specific IRF8 knockout resulted in deteriorated cardiac hypertrophy and fibrosis in response to pressure overload, as evidenced by higher ratios of HW/BW, HW/TL and LW/BW; larger cross sectional areas of cardiomyocytes; and higher expression levels of fetal genes and fibrotic markers than those of the controls ( Supplementary Fig. 4d–k ). Echocardiographic results also showed remarkable cardiac dilation and dysfunction in IRF8-KO mice compared with control mice ( Supplementary Fig. 4l ). These data provide further evidence that the cardiac-specific deletion of IRF8 promotes cardiac hypertrophy upon pressure overload. IRF8 transgenic mice exhibit attenuated cardiac hypertrophy Next, we sought to evaluate whether elevated IRF8 levels in the heart would attenuate cardiac hypertrophy. To address this hypothesis, transgenic (TG) mice with cardiac-specific overexpression of IRF8 were generated using the α-MHC promoter ( Supplementary Fig. 5a ). Four germ lines of IRF8-TG mice were verified by western blot analysis ( Supplementary Fig. 5b ). Under basal conditions, all the IRF8-TG mice were healthy and showed no apparent cardiac morphological or pathological abnormalities ( Supplementary Table 1 ). We then selected transgenic line 10, which expressed the highest levels of IRF8, for further experiments. IRF8-TG mice and their WT littermates (referred to as ‘NTG’) were subjected to AB surgery or a sham operation and examined after 8 weeks. As expected, AB-induced cardiac hypertrophy was significantly attenuated in IRF8-TG mice, as evidenced by lower ratios of HW/BW, HW/TL and LW/BW than those in the NTG mice ( Fig. 4a–c ). Similarly, the cross sectional area of cardiomyocytes was reduced by ~28% in AB-operated TG mice compared with NTGs ( Fig. 4d,e , P< 0.05; statistical analysis was carried out by two-way analysis of variance with general linear model procedures using a univariate approach; n =8 mice per experimental group). IRF8 overexpression significantly inhibited AB-triggered cardiac dilation and dysfunction as determined by echocardiographic and hemodynamic measurements ( Fig. 4f–h and Supplementary Table 3 ). IRF8-TG mouse tissue consistently exhibited decreased PSR staining positivity in the interstitial and perivascular spaces, as well as decreased collagen volumes following chronic AB compared with NTGs ( Fig. 4i,j ). To clarify whether different IRF8 protein expression levels had the similar effects on cardiac hypertrophy, the transgenic line 5, which expressed medium IRF8 protein levels, was subjected to AB surgery. The results showed that transgenic line 5 and transgenic line 10 had similar phenotypes, as evidenced by comparable HW/BW, LW/BW and HW/TL ratios; cross sectional areas, LV collagen volumes; and cardiac function (LVEDd, LVESd, FS%) ( Supplementary Fig. 5c–g ). Together, these gain-of-function data indicate that IRF8 overexpression attenuates cardiac hypertrophy and fibrosis in response to chronic pressure overload. 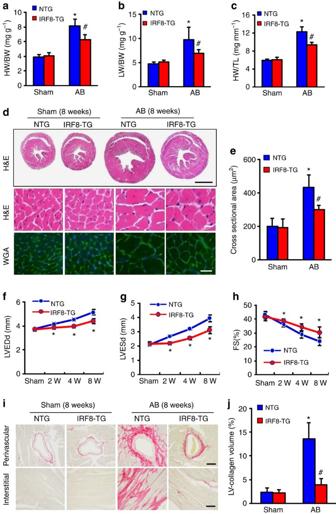Figure 4: Overexpression of IRF8 attenuates pressure overload-induced cardiac hypertrophy. (a–c) Statistical results for the ratios of (a) HW/BW, (b) LW/BW and (c) HW/TL in the indicated groups (n=13-16 mice per experimental group). (d) Histological analyses of the HE staining and WGA staining of NTG and TG mice 8 weeks after AB surgery (n=8 mice per experimental group; scale bar, 100 μm for upper HE staining, scale bar, 20 μm for lower HE staining and WGA staining). (e) Statistical results for the cell sectional area (n≥100 cells per experimental group). (f–h) f, The left ventricular end-diastolic dimension (LVEDd); g, the left ventricular end-systolic dimension (LVESd); h, FS% in NTG and TG mice from 2 to 8 weeks after AB surgery (n=6–8 mice per experimental group). (i) PSR staining on histological sections of the LV in the indicated groups 8 weeks after AB (n=8 mice per experimental group; scale bar, 50 μm). (j) Statistical results for LV collagen volume (n≥25 fields per experimental group). *P<0.05 versus NTG/sham; #P<0.05 versus NTG/AB. The data represent as the mean±s.d. Statistical analysis was carried out by two-way analysis of variance with general linear model procedures using a univariate approach. Figure 4: Overexpression of IRF8 attenuates pressure overload-induced cardiac hypertrophy. ( a – c ) Statistical results for the ratios of ( a ) HW/BW, ( b ) LW/BW and ( c ) HW/TL in the indicated groups ( n =13-16 mice per experimental group). ( d ) Histological analyses of the HE staining and WGA staining of NTG and TG mice 8 weeks after AB surgery ( n =8 mice per experimental group; scale bar, 100 μm for upper HE staining, scale bar, 20 μm for lower HE staining and WGA staining). ( e ) Statistical results for the cell sectional area ( n ≥100 cells per experimental group). ( f–h ) f, The left ventricular end-diastolic dimension (LVEDd); g, the left ventricular end-systolic dimension (LVESd); h, FS% in NTG and TG mice from 2 to 8 weeks after AB surgery ( n =6–8 mice per experimental group). ( i ) PSR staining on histological sections of the LV in the indicated groups 8 weeks after AB ( n =8 mice per experimental group; scale bar, 50 μm). ( j ) Statistical results for LV collagen volume ( n ≥25 fields per experimental group). * P< 0.05 versus NTG/sham; # P< 0.05 versus NTG/AB. The data represent as the mean±s.d. Statistical analysis was carried out by two-way analysis of variance with general linear model procedures using a univariate approach. Full size image IRF8 directly interacts with and inhibits NFATc1 Increasing evidence has suggested that numerous transcription factors or regulator factors are involved in the development of cardiac hypertrophy [4] , [7] . Therefore, we next sought to determine whether IRF8 would interfere with these hypertrophy-related transcription factors in hearts in response to pressure overload. To this end, we performed dual-luciferase reporter analysis using a Cignal 45-Pathway Reporter Array (SABiosciences, Cat number: CCA-901L), which provides comprehensive screening for measuring the activities of diverse transcription factors. Our initial results showed that NFATc1 transcriptional activity was dramatically inhibited by IRF8 in cardiomyocytes ( Supplementary Fig. 6a ). To validate this result further, NRCMs were co-infected with AdNFATc1-Luc and either AdIRF8 or AdshIRF8. These experiments clearly showed that NFATc1 activity was significantly limited by the overexpression of IRF8 but was increased significantly after IRF8 knockdown ( Supplementary Fig. 6b ). We also performed the luciferase reporter analysis in the hearts of IRF8-TG or -KO mice containing the NFAT-luciferase reporter gene and obtained similar results ( Fig. 5a,b ). 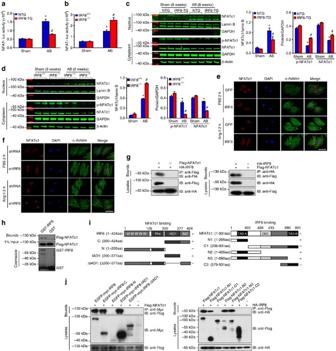Figure 5: IRF8 directly interacts with and inhibits nfatc1. (a,b) NFAT-luciferase activity in the hearts of (a) IRF8-TG or (b) IRF8−/−mice containing the NFAT-luciferase reporter gene (n=6 mice per experimental group). (c,d) Left: Representative western blots; right: quantitative results showing the total protein levels of NFATc1 in the nucleus and the phosphorylation and total protein levels of NFATc1 in the cytoplasm of IRF8-TG mice 8 weeks after AB surgery (c) or IRF8-KO mice 2 weeks after AB surgery (d). (e,f) Representative immunofluorescent stained images of NFATc1 in H9C2 cells transfected with IRF8 (e) or with shIRF8 (f), (red: NFATc1, blue: nuclear, green: α-actinin; scale bar, 50 μm). (g) Left: western blot performed with a Flag or HA antibody after co-IP of NFATc1 from HEK293T whole-cell lysates using a Flag antibody. Right: Western blot performed with a Flag or HA antibody after co-IP of IRF8 from HEK293T whole-cell lysates using an HA antibody. (h) Western blot analysis of a GST pull-down assay with lysates from Rosetta (DE3)Escherichia coliexpressing an exogenous GST fusion IRF8 protein (GST-IRF8) incubated with Flag-NFATc1-transfected HEK293T cell lysates. (i) Schematic representation of the full-length and truncated forms of IRF8 (left) and the full-length and truncated versions of NFATc1 (right) for determining the domain mediated their two interaction. (j) Left: Representative western blots performed using a Flag or Myc antibody after co-IP of the full-length and truncated forms of IRF8 from HEK293T whole-cell lysates using the Myc antibody; right: western blot performed with a Flag or HA antibody after co-IP of the full-length and truncated versions of NFATc1 from HEK293T whole-cell lysates using a Flag antibody. Three independent experiments were performed. *P<0.05 versus NTG or IRF8+/+/Sham, #P<0.05 versus NTG or IRF8+/+/AB. The data represent as the mean±s.d. Statistical analysis was carried out by two-way analysis of variance with general linear model procedures using a univariate approach. Figure 5: IRF8 directly interacts with and inhibits nfatc1. ( a , b ) NFAT-luciferase activity in the hearts of ( a ) IRF8-TG or ( b ) IRF8 −/− mice containing the NFAT-luciferase reporter gene ( n =6 mice per experimental group). ( c , d ) Left: Representative western blots; right: quantitative results showing the total protein levels of NFATc1 in the nucleus and the phosphorylation and total protein levels of NFATc1 in the cytoplasm of IRF8-TG mice 8 weeks after AB surgery ( c ) or IRF8-KO mice 2 weeks after AB surgery ( d ). ( e , f ) Representative immunofluorescent stained images of NFATc1 in H9C2 cells transfected with IRF8 ( e ) or with shIRF8 ( f ), (red: NFATc1, blue: nuclear, green: α-actinin; scale bar, 50 μm). ( g ) Left: western blot performed with a Flag or HA antibody after co-IP of NFATc1 from HEK293T whole-cell lysates using a Flag antibody. Right: Western blot performed with a Flag or HA antibody after co-IP of IRF8 from HEK293T whole-cell lysates using an HA antibody. ( h ) Western blot analysis of a GST pull-down assay with lysates from Rosetta (DE3) Escherichia coli expressing an exogenous GST fusion IRF8 protein (GST-IRF8) incubated with Flag-NFATc1-transfected HEK293T cell lysates. ( i ) Schematic representation of the full-length and truncated forms of IRF8 (left) and the full-length and truncated versions of NFATc1 (right) for determining the domain mediated their two interaction. ( j ) Left: Representative western blots performed using a Flag or Myc antibody after co-IP of the full-length and truncated forms of IRF8 from HEK293T whole-cell lysates using the Myc antibody; right: western blot performed with a Flag or HA antibody after co-IP of the full-length and truncated versions of NFATc1 from HEK293T whole-cell lysates using a Flag antibody. Three independent experiments were performed. * P< 0.05 versus NTG or IRF8 +/+ /Sham, # P< 0.05 versus NTG or IRF8 +/+ /AB. The data represent as the mean±s.d. Statistical analysis was carried out by two-way analysis of variance with general linear model procedures using a univariate approach. Full size image It is well recognized that the dephosphorylation and subsequent nuclear translocation of NFATc1 are important for NFAT-mediated transcriptional activation [24] . We therefore determined whether IRF8 affects the dephosphorylation and translocation of NFATc1. Nuclear NFATc1 levels in IRF8-TG and IRF8 knockout animals subjected to AB were determined by western blot ( Fig. 5c,d ). Compared with their respective controls, AB-induced nuclear translocation of NFATc1 was significantly blocked by IRF8 overexpression but was markedly increased by IRF8 deficiency ( Fig. 5c,d ). In support of these results, the AB-triggered reduction of phosphorylated and total NFATc1 in the cytoplasm was significantly lower in NTG hearts compared with IRF8-TG hearts ( Fig. 5c ). In contrast, the levels of phosphorylated and total NFATc1 in the cytoplasm were more reduced in AB-treated IRF8 −/− hearts than in control samples (IRF8 +/+ ) ( Fig. 5d ). Similar findings were also observed in AdIRF8- and AdshIRF8-infected NRCMs upon treatment with 1 μM of Ang II ( Supplementary Fig. 6c,d ). Furthermore, we confirmed these results by immunofluorescence analysis of H9C2 cells transfected with IRF8 or shIRF8 and of NRCMs infected with AdIRF8 or AdshIRF8 ( Fig. 5e,f and Supplementary Fig. 6e ). However, the nuclear NFATc2 and NFATc3 levels were increased in the IRF8 +/+ mice after the AB operation but there was no significant difference between the IRF8 knockout and IRF8 +/+ mice after AB surgery ( Supplementary Fig. 6f ). Based on these results, IRF8 negatively regulates the AB-induced dephosphorylation and subsequent nuclear translocation of NFATc1. The regulation of NFATc1 activity by IRF8 prompted us to ask whether IRF8 could directly interact with NFATc1. To answer this question, we transfected Flag-tagged NFATc1 and HA-tagged IRF8 into HEK293T cells and then performed co-immunoprecipitation (IP) experiments. The results showed that IRF8 precipitated with NFATc1 and vice versa ( Fig. 5g ). To confirm this interaction further, we performed a glutathione S -transferase (GST)-pull-down assay with GST-tagged IRF8. As expected, NFATc1 was eluted along with IRF8 ( Fig. 5h ). Then, we performed co-IP for endogenous protein interactions after extracting the proteins of NRCMs. Similar results were observed in NRCMs under basal conditions ( Supplementary Fig. 6g ). To exclude the possibility that IRF8/NFATc1 binding was artificially created during the process of IP and pull-down, we sought to identify their sub-cellular localization in H9C2 cells by immunofluorescent staining and observed that IRF8 and NFATc1 co-localized within cytoplasm ( Supplementary Fig. 6h ). Together, these results indicate that IRF8 physically interacts with NFATc1. Next, we sought to determine the region within IRF8 responsible for its binding to NFATc1 utilizing various deletion mutants of IRF8. Deletions of the amino-terminal 200 amino acids (N/1-200) and carboxy-terminal 47 amino acids (AID/377-424) did not affect the interaction of IRF8 with NFATc1. In contrast, this interaction was abolished by the deletion of amino acid 200 to 377 (N/1-200 and ΔIAD1/Δ200-377) (left panels of Fig. 5i,j ), indicating that the IRF-associated domain (IAD1:200-377aa) is a bona fide region of IRF8 that binds to NFATc1. Similarly, we generated a series of NFATc1 deletion mutants and mapped their ability to interact with IRF8. We found that two regions from amino acid 205 to the carboxyl terminus (C1/206-931 and C2/579-931) were not required for this interaction, whereas the TAD-A containing amino-terminal (N1/1-205, N2/1-426 and N3/1-690) was capable of binding to IRF8 (right panels of Fig. 5i,j ). Collectively, these results demonstrate an authentic interaction between IRF8 and NFATc1 that might underpin the negative regulation of NFATc1 by IRF8. To determine further whether such an interaction affected NFATc1 activity, we examined the effects of IRF8 on the luciferase activity of the established NFATc1-dependent genes including BNP, MCIP1.4 and EDN-1 (all of which are involved in cardiac hypertrophy) in AdshRNA/AdshIRF8 and AdGFP/AdIRF8-infected primary cultured cardiomyocytes. We found that IRF8 markedly inhibited BNP, MCIP1.4 and EDN-1 promoter activities, indicating that IRF8 recruited NFATc1 and then negatively regulated NFATc1-dependent transcriptional activity and blocked cardiac hypertrophy ( Supplementary Fig. 6i,j ). Furthermore, we generated a plasmid pcDNA3-IRF8ΔIAD1, in which the binding region (200–377 aa) was deleted, and encompassed by replication-defective adenoviral vectors. Then, NRCMs were co-infected with AdIRF8ΔIAD1 and the NFATc1-luciferase reporter. IRF8-mediated inhibition of NFATc1 was abolished by the deletion of IAD1 (200–377 aa) ( Supplementary Fig. 6k ). We also overexpressed IRF8ΔIAD1 in NRCMs, followed by the addition of Ang II to induce cell hypertrophy and we observed that Ang II-induced cell hypertrophy was dramatically suppressed by the overexpression of full-length IRF8 ( Supplementary Fig. 6l ). However, such inhibitory effects were completely lost in AdIRF8ΔIAD1-infected myocytes ( Supplementary Fig. 6l ). Together, these data suggest that the IAD1 region is essential for the IRF8-elicited inhibition of NFATc1 and, consequently, cell hypertrophy. IRF8-mediated pathological hypertrophy requires NFATc1 To determine whether NFATc1 signalling plays a causative role in the IRF8-mediated inhibition of cardiac hypertrophy, VIVIT (an inhibitor of NFAT) was infused into IRF8 +/+ and IRF8 −/− mice for 2 weeks via an Alzet 1002 osmotic minipump. Infused saline of a similar volume served as the control. These mice subsequently underwent treatment with AB for 2 weeks. Pre-treatment with VIVIT dramatically attenuated AB-induced cardiac remodelling in IRF8 +/+ mice ( Fig. 6a–f and Supplementary Table 4 ), consistent with previous reports [25] . Significantly, VIVIT treatment limited the aggravated effects of a IRF8-null mutation on cardiac remodelling in response to 2 weeks of AB, as evidenced by the following: lower ratios of HW/BW, LW/BW and HW/TL ( Fig. 6d–f ); smaller cross sectional areas of cardiomyocytes ( Fig. 6a,b ); and smaller collagen volumes ( Fig. 6a,c ) than those of saline-treated IRF8 −/− mice. Pre-treatment with VIVIT significantly abolished AB-induced increases in mRNA levels of hypertrophic and fibrotic markers, including ANP, BNP, β-MHC, CTGF, Collagen I and Collagen III, in IRF8 −/− mice compared with saline-treated animals ( Supplementary Fig. 7a,b ). These findings suggest that pre-inhibition of NFAT signalling protects against pressure overload-induced cardiac abnormalities in IRF8 −/− mice. 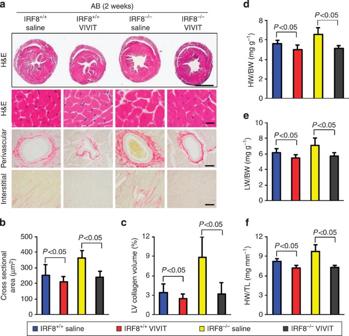Figure 6: Inhibition of NFATc1 abolishes abnormalities in IRF8−/−mice in response to pressure overload. (a) Histological analyses of HE staining and PSR staining of the indicated groups at 2 weeks after AB surgery and treated with VIVIT (n=5–8 mice per experimental group; scale bar, 100 μm for upper HE staining, scale bar, 20 μm for lower HE staining, scale bar, 50 μm for PSR staining). (b–f) Statistical results for the ratios of (b) cell sectional area (n≥100 cells per experimental group); (c) LV collagen volume (n≥25 fields per experimental group); (d) HW/BW; (e) LW/BW; and (f) HW/TL (n=11 mice per experimental group) in the indicated groups 2 weeks after AB surgery and treatment with VIVIT. The data represent as the mean±s.d. Statistical analysis was carried out by two-way analysis of variance with general linear model procedures using a univariate approach. Figure 6: Inhibition of NFATc1 abolishes abnormalities in IRF8 −/− mice in response to pressure overload. ( a ) Histological analyses of HE staining and PSR staining of the indicated groups at 2 weeks after AB surgery and treated with VIVIT ( n =5–8 mice per experimental group; scale bar, 100 μm for upper HE staining, scale bar, 20 μm for lower HE staining, scale bar, 50 μm for PSR staining). (b–f) Statistical results for the ratios of ( b ) cell sectional area ( n ≥100 cells per experimental group); ( c ) LV collagen volume ( n ≥25 fields per experimental group); ( d ) HW/BW; ( e ) LW/BW; and ( f ) HW/TL ( n =11 mice per experimental group) in the indicated groups 2 weeks after AB surgery and treatment with VIVIT. The data represent as the mean±s.d. Statistical analysis was carried out by two-way analysis of variance with general linear model procedures using a univariate approach. Full size image The above findings suggested that cardiac NFATc1 signalling activation neutralizes the protective effects of IRF8 on cardiac hypertrophy. To test this hypothesis, transgenic mice with a floxed CaNFATc1 were mated with transgenic αMHC-MerCreMer (MEM) mice to generate conditional CaNFATc1 transgenic mice (CaNFATc1-TG) ( Supplementary Fig. 8a ). These inducible CaNFATc1-TG mice were crossed with IRF8-TG mice to yield IRF8/CaNFATc1 double transgenic (DTG) mice ( Supplementary Fig. 8b ). Transgenic founders were identified by western blot analysis ( Supplementary Fig. 8c ). Mice (CaNFATc1-TGs and DTGs) at 6 weeks of age were subjected to tamoxifen (80 mg kg −1 per day, intraperitoneal injection) for 5 consecutive days to induce Cre-dependent recombination. We found that constitutive activation of NFATc1 promoted more AB-induced cardiac remodelling compared with MEM-Cre controls ( Fig. 7a–f and Supplementary Table 5 ). Remarkably, IRF8-mediated inhibition of cardiac hypertrophy was blocked by NFATc1 re-activation, which was evidenced by higher ratios of HW/BW, HW/TL and LW/BW in AB-treated DTG mice relative to AB-operated IRF8-TG mice ( Fig. 7d–f ). In addition, 4 weeks after AB, DTG hearts displayed larger cross sectional areas of cardiomyocytes and volumes of cardiac fibrosis than did IRF8-TG hearts ( Fig. 7a–c ). Markers of cardiac hypertrophy (ANP, BNP and β-MHC) and fibrosis (CTGF, Collagen I and Collagen III) were dramatically upregulated in DTG mice compared with IRF8-TG mice after 4 weeks after AB surgery ( Supplementary Fig. 8d,e ). Collectively, these results indicate that targeted NFATc1 activation negates the protective effects of IRF8 on cardiac hypertrophy in response to pressure overload. Thus, our findings suggest that IRF8 negatively modulates pathological cardiac remodelling, at least in part by inhibiting NFATc1 signalling. 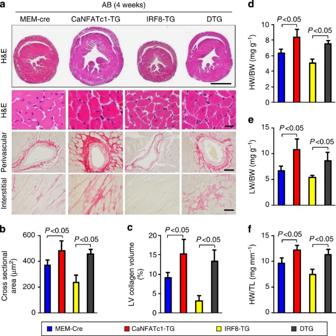Figure 7: Activation of NFATc1 negates the protective effects of IRF8 on cardiac hypertrophy in IRF8-TG mice. (a) Histological analyses of the HE and PSR staining of the indicated groups at 4 weeks after AB surgery (n=5–7 mice per experimental group; scale bar, 100 μm for upper HE staining, scale bar, 20 μm for lower HE staining, scale bar, 50 μm for PSR staining). (b–f) Statistical results for the ratios of (b) cell sectional area (n≥100 cells per experimental group); (c) LV collagen volume (n≥25 fields per experimental group); (d) HW/BW; (e) LW/BW; and (f) HW/TL (n=11 mice per experimental group) in the indicated groups at 4 weeks after AB surgery. The data represent as the mean±s.d. Statistical analysis was carried out by two-way analysis of variance with general linear model procedures using a univariate approach. Figure 7: Activation of NFATc1 negates the protective effects of IRF8 on cardiac hypertrophy in IRF8-TG mice. ( a ) Histological analyses of the HE and PSR staining of the indicated groups at 4 weeks after AB surgery ( n =5–7 mice per experimental group; scale bar, 100 μm for upper HE staining, scale bar, 20 μm for lower HE staining, scale bar, 50 μm for PSR staining). ( b – f ) Statistical results for the ratios of ( b ) cell sectional area ( n ≥100 cells per experimental group); ( c ) LV collagen volume ( n ≥25 fields per experimental group); ( d ) HW/BW; ( e ) LW/BW; and ( f ) HW/TL ( n =11 mice per experimental group) in the indicated groups at 4 weeks after AB surgery. The data represent as the mean±s.d. Statistical analysis was carried out by two-way analysis of variance with general linear model procedures using a univariate approach. Full size image IRF8 plays an important role in various organs, including the heart. However, its functional role in the development of cardiac hypertrophy and failure has remained unclear. In the present study, we utilized both gain-of-function and loss-of-function approaches to decipher thoroughly the role of IRF8 in chronic pressure overload-induced cardiac remodelling. Our findings demonstrate that an elevation in IRF8 is instrumental for hearts to resist pressure overload-induced hypertrophy and dysfunction and that conversely, the loss of IRF8 leads to exaggerated cardiac remodelling in response to hypertrophic stimuli. To our knowledge, this report is the first to identify IRF8 as a negative regulator of pathological cardiac hypertrophy. In past decades, genetically modified animal models have identified numerous pro-hypertrophic signalling pathways [4] , [26] . These pathways activate various transcriptional factors, driving expression of fetal cardiac and stress response genes and resulting in pathological cardiac hypertrophy [4] . Thus far, the best known of these transcriptional factors associated with cardiac hypertrophy are members of the NFAT family, including NFATc1, NFATc2, NFATc3 and NFAT5 (ref. 27) [27] . Generally, NFAT transcription factors are hyperphosphorylated and sequestered in the cytoplasm. Once dephosphorylated by activated calcineurin (CaN), NFATs rapidly translocate to the nucleus, where they work in coordination with other transcription factors to activate downstream targets [24] . Various genetic approaches have been applied to demonstrate the importance of the NFAT signalling pathway in the regulation of cardiac hypertrophy [28] . For example, cardiac-specific activation of NFAT by the constitutively active calcineurin catalytic subunit was shown to induce massive cardiac hypertrophy that quickly transitioned to heart failure and death in mice [29] . Conversely, the genetic inhibition of NFAT by different transgenic approaches (that is, overexpression of the calcineurin inhibitors Cabin1/Cain, AKAP79, MCIP1 and dnCaN) was shown to attenuate the hypertrophic response to a wide variety of acute stimuli in vivo [30] , [31] , [32] . Thus, molecules that selectively inhibit NFAT activation can be of great therapeutic interest in the treatment of cardiac hypertrophy. The identification of NFATc1 as an IRF8-interacting protein in the present study provides mechanistic insight into the relationship between IRF8 deficiency/overexpression and NFATc1 activation pertaining to cardiac hypertrophic states. Whereas cardiac IRF8 overexpression hampered NFATc1 nuclear translocation, IRF8 deficiency facilitated NFATc1 activation, providing evidence of the inhibitory effect of IRF8 on NFATc1. Such findings are consistent with a previous study that showed that IRF8 acts as a modifier of NFAT in osteoclast precursors [14] . Furthermore, activation of NFATc1 by the overexpression of its constitutively active form negated the protective effects of IRF8 on cardiac hypertrophy in mice; whereas the suppression of NFATc1 by VIVIT, a selective peptide inhibitor, prevented abnormalities in IRF8-null mice in response to pressure overload. However, upon AB surgery, IRF8/CaNFATc1 DTG mice still exhibited a reduced hypertrophic response compared with CaNFATc1-TG mice ( Fig. 7 and Supplementary Fig. 8 ). Thus, the inhibitory effects of IRF8 on cardiac hypertrophy might not be dependent only on the blocking of NFATc1 signalling. Based on our finding that IRF8 expression was significantly downregulated in DCM and HCM human hearts and hypertrophic murine hearts, we speculate that elevating the IRF8 level might represent a new strategy for treating hypertrophic heart disease that is worthy of additional validation and investigation. We further provide evidence that IRF8 physically interacts with NFATc1, which might render it inaccessible to activation by upstream phosphatases (that is, CaN) or kinases (that is, GSK). Intriguingly, we found that the IRF-associated domain (IAD1:200–377 aa) was required for IRF8 to inhibit NFATc1 activity. Our findings presented here suggest that the 200–377 aa of IRF8 involved in binding to NFATc1 might constitute a novel peptide inhibitor of NFATc1. However, future studies will be necessary to specify the active domain of IAD1 involved in blocking NFATc1 activity, and to determine its therapeutic potential for limiting pathological cardiac remodelling. Notably, parameters of cardiac function are similar among IRF8 +/+ , IRF8 −/− , NTG and IRF8-TG mice ( Supplementary Table 1 ). Thus, the IRF8 gene expression pattern appears to not affect myocardial contractile function under basal conditions. However, upon AB, wild-type mice (NTG and IRF8 +/+ ) developed cardiac hypertrophy and eventually heart failure, whereas IRF8-TG mice exhibited an attenuation of cardiac hypertrophy and thereby avoided cardiac dysfunction. Therefore, our results indicate that IRF8 might regulate cardiac function under pathological conditions. Interferon regulatory factors (IRFs) constitute a family of regulator factors comprising nine members (IRF1-9) in mammalian cells [9] . Previous studies have revealed the versatile and critical functions performed by this family in many biological processes [9] , [16] . Once activated, the IRFs shape the appropriate response by stimulating an overlapping but distinct set of target genes [33] . The cooperation or competition of different transcription factors of the IRF family at the DNA-binding level has been demonstrated in in vitro studies [34] , [35] , [36] . It is therefore possible that interplay exists among these different IRFs in the development of cardiac hypertrophy. Our recent findings showed that IRF3 and IRF9 protected against pressure overload-induced hypertrophic response by inactivating ERK1/2 or myocardin, respectively [37] , [38] , whereas IRF4 aggravated pressure overload-induced cardiac hypertrophy by activating the transcription of CREB in the heart [5] . In the present study, we demonstrated that IRF8 inhibited pressure overload-induced cardiac hypertrophy by interacting with NFATc1 to prevent NFATc1 nuclear translocation. Importantly, recent studies have also shown that there is cross-talk, including cross-inhibition or cross-activation among NFAT, myocardin, CREB and ERK signalling during cardiac hypertrophy [39] , [40] , [41] , [42] , [43] . These exciting cross-talk changes that occur during cardiac hypertrophy are of great significance because proper regulation of different pathways in the context of elaborate and highly complex signalling networks within the cell is strongly dependent on communication with other signalling molecules, resulting in either synergistic or antagonistic relationships that produce a spectrum of biological outcomes. Understanding the nature of cross-talk between these signalling pathways is indeed a major hurdle to understanding the molecular basis of the roles of the IRF family in cardiac remodelling. In conclusion, our present work provides both in vitro and in vivo evidence that IRF8 functions as a novel negative regulator factor of pathological cardiac hypertrophy. The mechanisms underlying IRF8-elicited cardioprotective effects are associated with direct inhibition of NFATc1 signalling, which suppresses the hypertrophic response caused by chronic pressure overload. These observations also provide new insights into the mechanisms of cardiac hypertrophy and could have significant implications for the development of novel strategies for the treatment of pathological cardiac hypertrophy by targeting IRF8. Reagents Antibodies against β-MHC (β-MHC, sc53090, 1:200 dilution), ANP (sc20158, 1:200 dilution), Lamin B (sc6217, 1:200 dilution), IRF8 (sc13043, 1:200 dilution), NFATc1 (sc13033, 1:200 dilution) and p-NFATC1 ser259 (sc32979, 1:200 dilution) were purchased from Santa Cruz Biotechnology (Dallas, TX, USA). The GAPDH antibody (MB001, 1:10,000 dilution) was ordered from Bioworld Technology (Harrogate, UK). Antibodies against HA (H6908, 1:1,000 dilution) and Flag (F3165, 1:1,000 dilution) were obtained from Sigma (St. Louis, MO, USA). The antibody against Myc (11814150001, 1:1,000 dilution) was obtained from Roche (Mannheim, Germany). The NFAT inhibitor VIVIT (480402) was purchased from Millipore (Billerica, MA, USA). The BCA protein assay kit came from Pierce (Rockford, IL, USA). We used IRDye 800CW-conjugated secondary antibodies (LI-COR Biosciences, Lincoln, NE, USA) for visualization. Fetal calf serum was ordered from Hyclone (Waltham, MA, USA). Cell culture reagents and all other reagents were purchased from Sigma (St. Louis, MO, USA). Plasmids The EGFP-myc-IRF8 recombinant plasmid was constructed by cloning the entire coding region of mouse IRF8 into the Eco RI and Xho I sites of the pEGFP-myc-C1 plasmid. HA-IRF8 was PCR amplified from the cDNA of HEK293T cells using the IRF8-5′ and IRF8-3′ primers. The IRF8 truncates, consisting of residues 200 to 424aa, 1 to 200aa and 200 to 377aa, were PCR amplified from HA-IRF8, using the IRF8-C-5′ and IRF8-3′, IRF8-5′ and IRF8-N-3′, IRF8-C-5′ and IRF8-IAD1-3′ primers, respectively. IRF8 deletion mutant lacking residues 200–377aa was generated by a one-step PCR-based mutagenesis procedure using EGFP-myc-IRF8 as the template. EGFP-myc-IRF8 was amplified with IRF8-dIAD1-5′ and IRF8-dIAD1-5′. The PCR products were phosphorylated with T4 PNK and then ligated to generate EGFP-myc-IRF8Δ200–377. The Flag-NFATc1 and EGFP-myc-NFATc1 constructs were generated by amplifying the NFATc1 gene-coding region with primers NFATc1-5′ and NFATc1-3′ from HA-NFATc1, and then they were subcloned into the plasmids psi-Flag-C1 and psi-EGFP-myc-C1. The NFATc1 fragments, consisting of residues 1 to 205aa, 206 to 931aa, 1 to 426aa, 1 to 690aa and 579 to 931aa, were PCR amplified using the NFATc1-5′ and NFATc1-N1-3′, NFATc1-C1-5′ and NFATc1-3′, NFATc1-5′ and NFATc1-N2-3′, NFATc1-5′ and NFATc1-N3-3′ and NFATc1-C2-5′ and NFATc1-3′ primers from Flag-NFATc1, respectively. The products were digested with Bam HI and Xho I and ligated into psi-Flag-C1 to create an in-frame fusion with Flag. pmCherry-IRF8 and GST-IRF8 constructs were generated by amplifying the IRF8 gene-coding region with primers IRF8-5′ and IRF8-3′ from HA-IRF8, followed by subcloning into pmCherry-C2 and pGEX-4T-1. The primers for these constructs are showed in Supplementary Table 6 . All plasmids were verified by sequencing. Animals used for study All the experiments involving animals were approved by the Animal Care and Use Committee of Renmin Hospital of Wuhan University. The following animals were used in this study. IRF8 −/− and cardiac-specific IRF8 transgenic mice. Full-length mouse IRF8 cDNA (Origene, MC200891) was cloned downstream of the cardiac α-myosin heavy chain (α-MHC) promoter. The linearized α-MHC-IRF8 plasmid was microinjected into fertilized mice embryos to produce cardiac-specific IRF8-TG mice identified by PCR analysis of tail genomic DNA. The PCR primers were as follows: forward: 5′-ATCTCCCCCATAAGAGTTTGAGTC-3′, and reverse: 5′-CCCACCAGTCAGGGAGGAT-3′. Four independent TG lines were established and studied. IRF8 knockout mice (IRF8 −/− , B6.129P2-Irf8 tm1Hor /Kctt) were purchased from the European Mouse Mutant Archive (EMMA, EM: 02414). The IRF8 −/− mice were crossed with C57BL/6J mice to produce the F1 generation (IRF8 heterozygous), which was backcrossed with the C57BL/6J strain to obtain the F2 generation (IRF8 heterozygous) and then further backcrossed to the C57BL/6J background until the F9 generation (IRF8 heterozygous). F9 generation male and female mice were crossed with each other to produce IRF8 −/− mice (pure C57BL/6J background). IRF8-Flox mice (B6(Cg)-Irf8 tm1.1Hm /J) were purchased from Jackson Laboratory (Stock No. : 014175). The male IRF8 −/− , IRF8 transgene and their wild-type littermates, aged 8–10 weeks old (with BWs of 24–27 g), were used in the described experiments. Cardiac-specific CaNFATc1-TG and CaNFATc1/IRF8DTG Mice. To obtain the CaNFATc1 flox mice, we subcloned an N-terminal hemagglutinin-tagged, C-terminal Flag-tagged CaNFATc1 containing serine to alanine substitutions in the conserved serine-rich domain and all three serine-proline repeats (NFATc-mSRD-mSPx3) into the CAG-CAT-LacZ construct, which contains a CMV enhancer and a chicken β-actin gene promoter, linked to the chloramphenicol acetyltransferase (CAT) gene and flanked by loxp sites. In this construct, CaNFATc1 expression is blocked by the presence of the CAT gene; when the CAT sequence is excised by Cre recombinase, CaNFATc1 is expressed. The CaNFATc1 flox mice were crossed with mice carrying the α-MHC–MerCreMer transgene (MEM-Cre-Tg (Myh6-cre/Esr1, Jackson Laboratory, 005650)) to yield CaNFATc1-Cre-TG mice. For cardiac-specific overexpression of CaNFATc1, tamoxifen (80 mg kg −1 per day, Sigma, T-5648) was injected for 5 consecutive days into MEM-Cre-TG (+) mice containing the CaNFATc1 gene at 6 weeks of age. The CaNFATc1-TG mice were identified by PCR analysis of tail genomic DNA using the following primers: forward: 5′-ATCTCCCCCATAAGAGTTTGAGTC-3′, and reverse: 5′-CAGGGTTGCTGTAGACG-3′. IRF8-TG mice were crossed with CaNFATc1-Cre-TG mice to breed CaNFATc1-Cre/IRF8 double transgenic (DTG) mice. MEM-Cre-TG mice served as the controls. All the experiments were performed in male mice aged 8–10 weeks old (BW 24–27 g). Cardiac-specific NFAT-luc TG mice. To determine the effect of IRF8 on the transcriptional activity of NFAT in vivo , NFAT-luc TG mice (B6; FVB-TG (Myh6/NFAT-luc)1 Jmol J −1 ) were ordered from Jackson Laboratory (013781) and were backcrossed as described above. Then, we crossed mice containing the cardiac-specific IRF8 transgene or IRF8 −/− mice with mice containing the NFAT-luciferase reporter transgene to produce cardiac-specific IRF8-TG or IRF8 −/− mice containing the NFAT-luciferase reporter gene. Mice were anesthetized using sodium pentobarbital (50 mg kg-, intraperitoneal, Sigma), and the adequacy of the anaesthesia was confirmed by the absence of a toe pinch reflex. All surgeries and subsequent analyses were performed in a blinded fashion. Aortic banding Cardiac hypertrophy mouse models were induced by AB [3] , [5] , [6] , [37] . Briefly, the left chest of each mouse was opened to identify the thoracic aorta by blunt dissection at the second intercostal space after anesthetization with pentobarbital sodium and the absence of any toe pinch reflex. We then performed AB using 7–0 silk sutures to band the thoracic aorta against a 27-gauge (BWs of 24–25 g) or 26-gauge (BWs of 26–27 g) needle. The needle was removed before closing the thoracic cavity. In addition, adequate constriction of the aorta was determined by Doppler analysis. A similar procedure, without constricting the aorta, was performed in the sham-operated group. Treatment of mice with VIVIT VIVIT, an NFAT inhibitor, was purchased from Millipore (480401). The VIVIT powder was dissolved in purified water and then filtered with a 0.22 μm membrane. VIVIT (10 mg kg −1 per day) was continuously infused over a 2-week period using an Alzet 1002 osmotic minipump implanted subcutaneously over the dorsal thorax. Echocardiography and hemodynamic measurements Echocardiography and hemodynamic measurements were performed at the indicated times after the mice were anesthetized using 1.5–2% isoflurane [3] , [5] , [6] , [22] , [37] , [44] , [45] . For echocardiography, M-mode images derived from the short axis of the LV were recorded using a Mylab30CV (ESAOTE) machine with a 15-MHz probe. To measure the LVEDD, LVESD and LVFS (LVFS (%)=(LVEDD-LVESD)/LVEDD × 100%), M-mode measurements of the LV internal diameter were obtained from at least three beats and then averaged. Cardiac catheterization studies were performed using a 1.4-French Millar catheter-tip micromanometer catheter (SPR-839; Millar Instruments), which was inserted through the right carotid artery into the left ventricle. The pressure and dp/dt were recorded continuously with an Aria pressure-volume conductance system coupled to a Powerlab/4SP A/D converter and were stored and displayed on a personal computer. Histological analysis Hearts were fixed in 10% formalin and embedded in paraffin using standard histological procedures. Subsequently, these hearts were sectioned transversely at 5 μm. Sections were stained with hematoxylin-eosin for histopathology or with PSR to evaluate collagen deposition. The myocyte cross sectional area was measured using a quantitative digital image analysis system (Image-Pro Plus, version 6.0) from images captured from FITC-conjugated wheat germ agglutinin (WGA, Invitrogen) stained sections. More than 100 myocytes in the sections were outlined in each group. Cultured NRCMs and recombinant adenoviral vectors Primary cultures of NRCMs were prepared according to the following protocol [3] , [5] , [6] . Briefly, PBS containing 0.03% trypsin and 0.04% collagenase type II was used to isolate cardiomyocytes from 1- to 2-day-old Sprague–Dawley rats. After removing fibroblasts by a differential attachment technique, NRCMs were seeded at a density of 2 × 10 5 cells per well onto six-well culture plates coated with gelatin in plating medium consisting of DMEM/F12 medium supplemented with 20% fetal calf serum, BrdU (0.1 mM, to inhibit the proliferation of fibroblasts) and penicillin/streptomycin. After 48 h, the culture medium was replaced with serum-free DMEM/F12 for 12 h prior to stimulation with angiotensin II (Ang II, 1 μM) or phenylephrine (PE, 100 μM). To overexpress IRF8, the entire coding region of the rat IRF8 gene, under control of the cytomegalovirus promoter, was encompassed by replication-defective adenoviral vectors. A similar adenoviral vector encoding the green fluorescent protein gene was used as a control. To knockdown IRF8 expression, three rat shIRF8 constructs were obtained from SABiosciences (KR59496G). The construct that decreased IRF8 levels to the greatest extent was selected for all further experiments. AdshRNA was the non-targeting control. NCRMs were infected with adenovirus in diluted media at a multiplicity of infection of 100 for 24 h. Immunofluorescence analysis The NRCMs was stained with α-actinin antibody to assess the cell surface area, and NFATc1 localization in H9C2 cells and NRCMs was determined by immunofluorescence staining. Briefly, cardiomyocytes were stimulated with 1 μM of Ang II for 48 h after infection with different adenoviruses for 24 h. The cells were then fixed with 3.7% formaldehyde in PBS for 15 min at room temperature, permeabilized with 0.1% Triton X-100 in PBS for 40 min and stained with α-actinin (1:100 dilution) using standard immunofluorescence staining techniques. The H9C2 cells were transfected with IRF8 or shIRF8 for 24 h and were subsequently stimulated with 1 μM of Ang II for 2 h. The procedure was the same as that used for cardiomyocytes staining with NFATc1 (1:50 dilution). Quantitative real-time PCR and western blotting Total mRNA was extracted from ventricles and primary cells using TRIZol reagent (Invitrogen), and cDNA was synthesized using oligo (dT) primers with the Transcriptor First Strand cDNA Synthesis Kit (Roche). Selected gene differences were confirmed by quantitative real-time PCR using SYBR green (Roche) and the results were normalized against GAPDH gene expression. The primers for real-time PCR are shown in Supplementary Table 7 . Total protein and nuclear protein were extracted from ventricles and primary cells, respectively [37] . The protein concentration was determined using the Pierce BCA Protein Assay kit (Pierce). Fifty micrograms of protein was used for SDS–PAGE (Invitrogen), and the proteins were transferred to a polyvinylidene fluoride membrane (Millipore), which were incubated with various primary antibodies overnight at 4 °C. After incubation with a secondary IRDye 800CW-conjugated antibody (Li-Cor Biosciences, at 1:10,000 dilution), signals were visualized with an Odyssey Imaging System (Li-Cor Biosciences). The specific protein expression levels were normalized to GAPDH for the total lysates or to Lamin B for the nuclear proteins on the same nitrocellulose membrane. Full gel scans are shown in Supplementary Fig. 9 . Luciferase reporter assays The luciferase reporter assay in vivo was performed according to the following protocol [28] , [46] , [47] . Briefly, mice expressing NFAT-Luc were euthanized with an overdose of pentobarbital solution (200 mg kg −1 intraperitoneal). The heart was isolated and lysed using tissue lysis buffer from Promega according to the manufacturer’s protocol. Next, the lysates were centrifuged for 20 min at 10,000 r.c.f., and the supernatant was used to determine both luciferase activity and protein content. Luciferase activity was measured using a Luciferase Assay System kit (Promega), and a Single-Mode SpectraMax Microplate Reader (Molecular Devices). Protein content was determined using the BCA protein assay kit, and this content was used to normalize luciferase activity per sample. Three copies of the NFATc1 binding site from the human IL -2 distal promoter linked to the luciferase gene were cloned into the pGL3-basic plasmid to obtain the NFATc1-luciferase reporter vector (p3 × NFATc1-luc). NRCMs were seeded onto 24-well plates at a density of 1 × 10 5 per well the day before infection. Either AdIRF8 or AdshIRF8 with AdNFATc1-Luc/BNP-Luc/MCIP1.4-Luc /EDN-1-Luc was co-infected into cardiomyocytes. After 24 h of stimulation with Ang II, the cells were harvested, washed three times with PBS and lysed in 100 μl passive lysis buffer (Promega) according to the manufacturer’s instructions. Cell debris was removed by centrifugation, and the supernatant was used for the luciferase assay with a Single-Mode SpectraMax Microplate Reader. A Cignal 45-Pathway Reporter Array (SABiosciences, CCA-901L) was used to rapidly identify relevant pathways for further analysis in H9C2 cells according to the manufacturer’s protocol. In brief, we added 200 ng of green fluorescent protein or IRF8 plasmid diluted in 50 μl Opti-MEM to each well of the Cignal Finder Array plate, and then we resuspended the reporter assay constructs by gently tapping the side of the plate. After setting the tubes at room temperature for 5 min, 0.6 μl of Attractene Transfection Reagent (Qiagen) in 50 μl of Opti-MEM was added to each well containing 50 μl of the diluted nucleic acids. After the 20-minute incubation for complex formation was completed, 50 μl of a prepared cell suspension (8 × 10 4 cells in Opti-MEM containing 10% fetal bovine serum, FBS) was added to each well containing the construct-Attractene complexes. After 16 h of transfection, the medium was changed to complete growth medium (DMEM with 10% FBS, 0.1 mM NEAA, 1 mM sodium pyruvate, 100 U ml −1 penicillin and 100 μg ml −1 streptomycin). Finally, 48 h after co-transfection, luciferase activity was determined using the Dual-Luciferase Reporter Assay System (Promega). Immunoprecipitation Cultured HEK293T cells co-transfected with the appropriate plasmids were collected and sonicated in an IP buffer (20 mM Tris-HCl (pH 8.0), 150 mM NaCl, 1 mM EDTA and 0.5% NP-40) supplemented with a protease inhibitor cocktail (Roche). After incubating for 20 minutes at 4 °C, followed by centrifuging 13,000 g for 15 min, the cell lysates were precleared with normal mouse or rabbit immunoglobulin G and protein A/G-agarose beads (11719394001, 11719386001, Roche) for 3 h at 4 °C. The precleared lysates (500 μl) were then incubated with 1 μg of antibody and 10 μl of protein A/G-agarose beads on a rocking platform at 4 °C overnight. The immunocomplex was collected, washed five to six times with cold IP buffer and blotted using the indicated primary antibodies. Co-IP for endogenous proteins was performed in the cytoplasmic protein of NRCMs isolated using an NE-PER nuclear and cytoplasmic extraction kit (Pierce, Cat number: 78835). GST pull-down assay The GST-IRF8 fusion protein was expressed in Rosetta (DE3) Escherichia coli and was purified and immobilized to glutathione-Sepharose 4B beads (GE healthcare Biosciences AB), according to the manufacturer’s instructions. In brief, the GST-IRF8 beads were incubated with Flag-NFATc1-transfected HEK293T cell lysates in IP buffer (20 mM Tris-HCl, pH 8.0, 150 mM NaCl, 1 mM EDTA and 0.5% NP-40 supplemented with protease inhibitor cocktail) for 4 h at 4 °C. The beads were then washed four times with IP lysis buffer in the absence of cocktail. Eluted bound proteins were resolved by SDS–PAGE and were analysed by western blot using anti-Flag antibodies. Confocal microscopy H9C2 cells were grown on coverslips in 24-well plates. After co-transfection with pmCherry-IRF8 and pEGFP-NFATc1 for 48 h, the cells were fixed using 4% fresh paraformaldehyde for 15 min, followed by three washes with PBS and 5 min of permeabilization with 0.2% Triton X-100 in PBS, followed by incubation in an Image-IT FX signal enhancer (I36933, Invitrogen) for 30 min. Subsequently, the cells were washed three times with TBST and were stained with DAPI (1 g ml −1 , 15 min). The slides were mounted with mounting solution (D2522, Sigma), and images were acquired using a confocal laser-scanning microscope (Fluoview 1000; Olympus). Human heart samples Samples of failing human hearts were collected from the left ventricles of DCM patients and HCM patients (Patient 1: male, 23 years old, interventricular septal thickness (IVS)=23 mm, ejection fraction (EF)=57%; Patient 2: male, 30 years old, IVS=20 mm, EF=66%; Patient 3: female, 40 years old, IVS=25 mm, EF=58%; Patient 4: male, 50 years old, IVS=31 mm, EF=74%) undergoing heart transplants [6] . Control samples were obtained from the left ventricles of normal heart donors who died in accidents but whose hearts were not suitable for transplantation for noncardiac reasons. Written informed consent was obtained from the families of prospective heart donors. All the procedures involving human samples conformed to the principles outlined in the Declaration of Helsinki and were approved by the Renmin Hospital of Wuhan University Review Board in Wuhan, China. Statistical analysis Data are represented as the mean±s.d. Student’s two-tailed t- test was used to compare the means of two groups of samples, and two-way analysis of variance with general linear model procedures using a univariate approach was applied for more than two groups. All statistical analyses were performed with SPSS software, version 13.0. Statistical significance was set at P< 0.05. How to cite this article : Jiang, D.-S. et al. IRF8 suppresses pathological cardiac remodelling by inhibiting calcineurin signalling. Nat. Commun. 5:3303 doi: 10.1038/ncomms4303 (2014).